Interstitial cells of Cajal integrate excitatory and inhibitory neurotransmission with intestinal slow-wave activity The enteric nervous system contains excitatory and inhibitory neurons, which control contraction and relaxation of smooth muscle cells as well as gastrointestinal motor activity. Little is known about the exact cellular mechanisms of neuronal signal transduction to smooth muscle cells in the gut. Here we generate a c-Kit CreERT2 knock-in allele to target a distinct population of pacemaker cells called interstitial cells of Cajal. By genetic loss-of-function studies, we show that interstitial cells of Cajal, which generate spontaneous electrical slow waves and thus rhythmic contractions of the smooth musculature, are essential for transmission of signals from enteric neurons to gastrointestinal smooth muscle cells. Interstitial cells of Cajal, therefore, integrate excitatory and inhibitory neurotransmission with slow-wave activity to orchestrate peristaltic motor activity of the gut. Impairment of the function of interstitial cells of Cajal causes severe gastrointestinal motor disorders. The results of our study show at the genetic level that these disorders are not only due to loss of slow-wave activity but also due to disturbed neurotransmission. The enteric nervous system contains two major classes of neurons: (1) excitatory neurons, which constitute the majority of neurons that make up functional circuits and are responsible for generating excitatory output, and (2) inhibitory neurons, which provide a rich variety of inhibitions that shape the output of functional circuits. Proper functioning of gastrointestinal (GI) motility critically depends on the interplay between excitatory and inhibitory enteric neurons, and on signalling to the smooth musculature [1] , [2] . Interstitial cells of Cajal (ICC) form a cellular network that is embedded in the musculature of the GI tract [3] , [4] , [5] , [6] . Previous studies provided clear evidence that ICC generate a rhythmic pacemaker current, which manifests itself as slow waves in the membrane potential of smooth muscle cells, resulting in rhythmic bowel contractions [4] , [7] , [8] . However, a role of ICC in the transmission of excitatory and inhibitory signals from enteric neurons to smooth muscle cells is highly controversial and remains an outstanding question [8] , [9] , [10] , [11] , [12] , [13] , [14] , [15] , [16] . This is mainly because of the general lack of models and systems to study ICC function in adult animals at genetic level [9] , [11] , [16] . Using genetic engineering in mice, we generated an inducible c-Kit CreERT2 knock-in allele, which enables, for the first time, genetic manipulation of ICC in vivo at defined time points during development and in adults. With the help of this novel model, we analysed ICC function in vivo by genetic loss-of-function studies. We show that ICC are essential for generation of slow waves and rhythmic contractions of the smooth musculature in adult animals. In addition, ICC integrate and mediate excitatory and inhibitory neurotransmission in the gut. These data provide the first in vivo genetic evidence that ICC integrate intestinal pacemaker activity with enteric neurotransmission to control and coordinate digestive activity in adult animals. As impaired ICC function causes severe GI motor disorders [17] , we provide genetic evidence that this is at least, in part, due to altered enteric neurotransmission. Time-specific genetic targeting of ICC in adult mice To test the hypothesis that enteric neurons signal via ICC to smooth muscle cells, it is imperative to target ICC in the gut. To achieve this, we took advantage of the exquisite fidelity of the inducible site-specific Cre/loxP recombination system [18] . We generated a CreER T2 allele as a knock-in at the endogenous c-Kit locus ( c-Kit CreERT2/+ mouse line; Supplementary Fig. S1a-d ). In this mouse line, Cre can be activated by tamoxifen (TAM) administration at defined time points in the c-Kit lineage during embryogenesis and in adult animals. c-Kit is a receptor tyrosine kinase, which is specifically expressed in ICC in the gut musculature ( Fig. 1a ), and c-Kit serves as the only well-established marker for ICC [4] , [7] , [17] . By crossing c-Kit CreERT2/+ mice with the switchable double-fluorescent R26 mT-mG/+ reporter mouse line [19] , we obtained c-Kit CreERT2/+ ; R26 mT-mG/+ mice ( Fig. 1b ), in which TAM-activatable CreER T2 was specifically expressed in ICC as manifested by enhanced green fluorescent protein expression of c-Kit-positive cells after TAM administration ( Fig. 1c and Supplementary Fig. S2 ). Quantification of enhanced green fluorescent protein/c-Kit double-positive cells revealed a TAM-induced recombination efficiency of ICC in the small and large intestine of >90% ( Fig. 1e ). 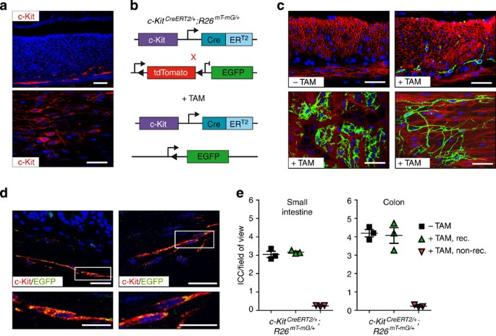Figure 1: Time-specific genetic manipulation of ICC. (a) Representative confocal microscopic images of c-Kit (red)-stained cryostat sections (upper panel) and whole mounts (lower panel) of murine colon. Scale bars, 50 μm. (b) Genetic strategy used to activate enhanced green fluorescent protein (EGFP) expression in ICC. (c) TAM-induced CreERT2-mediated EGFP expression (green) in small and large intestine. Animals were treated with TAM (+TAM) or vehicle (−TAM) for 3 days as indicated. Upper panel: colonic tissue sections. Lower panel: whole mounts from small intestine (left) and colon (right). Scale bars, 50 μm. (d) Representative images of c-Kit (red) immunofluorescence and TAM-induced EGFP (green) expression shows colabelling (yellow) of ICC in murine colon. Nuclei were counterstained with TOPRO-3 (blue). Scale bars, 50 μm for micrographs, 25 μm for high-magnification panels. (e) Quantification of +TAM-induced recombination of theR26mT-mGallele in c-Kit antibody-stained ICCs in the small intestine (left panel) and colon (right panel); rec., EGFP and c-Kit double-positive cells; non-rec., c-Kit single-positive cells. Vehicle-treated animals (−TAM) showed no recombination events (mean±s.e.m.;n=3 per group; 30 representative fields of view per mouse). Figure 1: Time-specific genetic manipulation of ICC. ( a ) Representative confocal microscopic images of c-Kit (red)-stained cryostat sections (upper panel) and whole mounts (lower panel) of murine colon. Scale bars, 50 μm. ( b ) Genetic strategy used to activate enhanced green fluorescent protein (EGFP) expression in ICC. ( c ) TAM-induced CreER T2 -mediated EGFP expression (green) in small and large intestine. Animals were treated with TAM (+TAM) or vehicle (−TAM) for 3 days as indicated. Upper panel: colonic tissue sections. Lower panel: whole mounts from small intestine (left) and colon (right). Scale bars, 50 μm. ( d ) Representative images of c-Kit (red) immunofluorescence and TAM-induced EGFP (green) expression shows colabelling (yellow) of ICC in murine colon. Nuclei were counterstained with TOPRO-3 (blue). Scale bars, 50 μm for micrographs, 25 μm for high-magnification panels. ( e ) Quantification of +TAM-induced recombination of the R26 mT-mG allele in c-Kit antibody-stained ICCs in the small intestine (left panel) and colon (right panel); rec., EGFP and c-Kit double-positive cells; non-rec., c-Kit single-positive cells. Vehicle-treated animals (−TAM) showed no recombination events (mean±s.e.m. ; n =3 per group; 30 representative fields of view per mouse). Full size image Acute ICC depletion disturbs GI motility To gain insights into the specific role of ICC for enteric neurotransmission, we crossed c-Kit CreERT2/+ mice with conditional LSL-R26 DTA/+ animals ( Fig. 2a ) [20] , which carry a latent diphteria toxin A (DTA) expression cassette. After 3 days of TAM treatment, we observed depletion of more than 50% of the ICC network in the gut ( Fig. 2b ). The ICC depletion resulted in a significantly disturbed GI motility with an increased total GI transit time of more than 5 h as measured by carmine red staining ( Fig. 2d ). Besides ICC, mast cells express c-Kit in the GI tract [21] . To exclude a role of mast cell depletion in our model system, we performed adaptive bone marrow transfer from wild-type (WT) animals into c-Kit CreERT2/+ ; LSL-R26 DTA/+ mice. Thereby, we were able to reconstitute these animals with WT mast cells ( Supplementary Fig. S3 ). To explore whether mast cells modulate GI motility, we treated c-Kit CreERT2/+ ; LSL-R26 DTA/+ mice, repopulated with WT mast cells, with TAM. Three days later, all animals showed a similar increased GI passage time as observed in TAM-treated c-Kit CreERT2/+ ; LSL-R26 DTA/+ animals ( Fig. 2e ). Thus, depletion of mast cells does not modulate GI motility in our experimental setup. 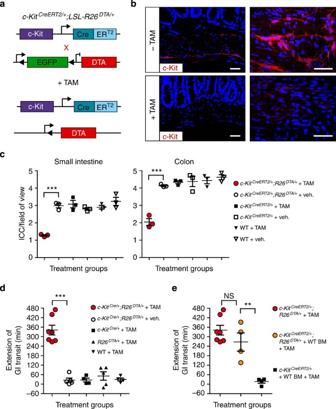Figure 2: Depletion of ICC results in disturbed GI motility. (a) Genetic strategy used to deplete ICC in adult animals by conditional expression of DTA. (b) Representative confocal microscopic images of cryostat sections (left panels) and whole-mounts (right panels) from c-Kit (red)-stained colon of vehicle (veh.; upper panels, −TAM)- and TAM (lower panels,+TAM)-treatedc-KitCreERT2/+;LSL-R26DTA/+mice. Nuclei were counterstained with TOPRO-3 (blue); scale bars, 50 μm. (c) Quantification of ICC in small intestine (left panel) and colon (right panel) after 3 days of +TAM or veh. treatment of indicated genotypes (n=3 per group; 30 representative fields of view per mouse; ***P<0.001; Studentst-test). (d) Extension of whole GI transit time after 3 days of +TAM or veh. treatment of the indicated genotypes (***P<0.001; Studentst-test). GI transit time was measured before and after treatment of each animal. (e) Extension of whole GI transit time of WT bone marrow (BM)-transplantedc-KitCreERT2/+;LSL-R26DTA/+and control mice treated with +TAM (N.S., not significant; **P<0.01; Studentst-test). All graphs represent mean±s.e.m. Figure 2: Depletion of ICC results in disturbed GI motility. ( a ) Genetic strategy used to deplete ICC in adult animals by conditional expression of DTA. ( b ) Representative confocal microscopic images of cryostat sections (left panels) and whole-mounts (right panels) from c-Kit (red)-stained colon of vehicle (veh. ; upper panels, −TAM)- and TAM (lower panels,+TAM)-treated c-Kit CreERT2/+ ; LSL-R26 DTA/+ mice. Nuclei were counterstained with TOPRO-3 (blue); scale bars, 50 μm. ( c ) Quantification of ICC in small intestine (left panel) and colon (right panel) after 3 days of +TAM or veh. treatment of indicated genotypes ( n =3 per group; 30 representative fields of view per mouse; *** P <0.001; Students t -test). ( d ) Extension of whole GI transit time after 3 days of +TAM or veh. treatment of the indicated genotypes (*** P <0.001; Students t -test). GI transit time was measured before and after treatment of each animal. ( e ) Extension of whole GI transit time of WT bone marrow (BM)-transplanted c-Kit CreERT2/+ ; LSL-R26 DTA/+ and control mice treated with +TAM (N.S., not significant; ** P <0.01; Students t -test). All graphs represent mean±s.e.m. Full size image ICC ablation disrupts intestinal slow-wave activity To determine the role of ICC for GI motility in distinct functional regions of the GI tract, we analysed gastric emptying and small bowel passage by fluorescence measurements and colonic motility, using the well-established colon bead expulsion test. The ICC depletion resulted in delayed gastric emptying and an extended small and large bowel passage time ( Fig. 3a–d ). This is consistent with observations in W/W v animals carrying a hypomorphic c-Kit allele in the germline [4] , [7] , [22] . These animals have a reduced ICC number and display a severely disturbed GI motility. Similar observations were made using c-Kit-blocking antibodies [23] , [24] . To determine whether disturbed GI motility in TAM-treated c-Kit CreERT2/+ ; LSL-R26 DTA/+ animals is due to disrupted slow-wave activity, we measured the electrical activity and contraction of the small intestinal smooth musculature ( Fig. 3e-i ). Control animals displayed typical ongoing rhythmic contractions, which are due to slow-wave-type electrical activity, whereas TAM-treated c-Kit CreERT2/+ ; LSL-R26 DTA/+ animals showed dysrhythmia due to uncoordinated spontaneous contractions and lack of slow-wave-type electrical activity ( Fig. 3e-i and Supplementary Fig. S4a ) as demonstrated before in W/W v animals [7] , [25] . This validates an essential role of ICC for the generation of slow waves also in acute ICC-depleted adult animals. 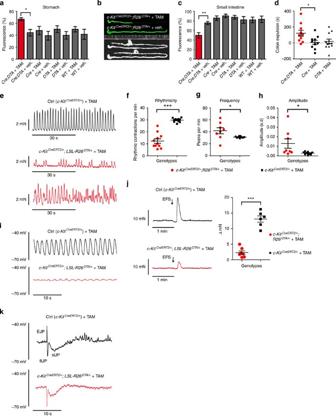Figure 3: Loss of slow-wave activity and excitatory neurotransmission in ICC-depleted animals. (a–c)In vivogastric emptying and small intestinal transit measured by quantification of indocyanin green (ICG) fluorescence. (a) Gastric emptying of indicated genotypes (n=3-4; *P<0.05; Studentst-test). (b) Representative image of small intestinal transit of ICG in TAM- and vehicle (veh.)-treated animals of indicated genotypes. (c) Small intestinal transit of indicated genotypes (n=3-4; **P<0.01; Studentst-test). (d) Change of colonic transitin vivomeasured by bead expulsion time before and after TAM treatment (n=10-11; *P<0.05; Studentst-test). (e)Ex vivomuscle strip recordings showing spontaneous mechanical activity of ileal circular smooth musculature from TAM-treated control (upper panel) andc-KitCreERT2/+;LSL-R26DTA/+animals (middle and lower panel, representative traces of two different animals). (f) Quantification of rhythmic contractions ine. The number of contractions with a regular distance between the peaks was counted (1 min of trace was analysed,n=11; ***P<0.001; Studentst-test). Frequency (g) and calculated s.d. of amplitude (h) of contractions in ileum preparations (1 min trace of each animal was analysed,n=8-9; *P<0.05; Studentst-test). (i) Intracellular microelectrode recordings display spontaneous electrical slow-wave activity in representative small intestinal circular smooth muscle cells from TAM-treated control animals (upper panel). Abolition of slow waves in TAM-treatedc-KitCreERT2/+;LSL-R26DTA/+mice (lower panel;n=3; recordings of 15 cells per animal). (j) Representative traces show contractile response of circular colonic muscle strips to EFS of TAM-treated control (upper left panel) andc-KitCreERT2/+;LSL-R26DTA/+(lower left panel) mice. Right panel: graph showing EFS-induced contraction force relative to the baseline before EFS (n=6-7; ***P<0.001; Studentst-test). (k) Representative intracellular microelectrode recordings of colonic circular smooth muscle cells of the indicated genotypes in response to EFS (n=3; recordings of 15 cells per animal). The EJP is lost in TAM-treatedc-KitCreERT2/+;LSL-R26DTA/+mice, whereas the fIJP and the sIJP remain unaffected by ICC depletion. All graphs show mean±s.e.m. Figure 3: Loss of slow-wave activity and excitatory neurotransmission in ICC-depleted animals. ( a – c ) In vivo gastric emptying and small intestinal transit measured by quantification of indocyanin green (ICG) fluorescence. ( a ) Gastric emptying of indicated genotypes ( n =3-4; * P <0.05; Students t -test). ( b ) Representative image of small intestinal transit of ICG in TAM- and vehicle (veh. )-treated animals of indicated genotypes. ( c ) Small intestinal transit of indicated genotypes ( n =3-4; ** P <0.01; Students t -test). ( d ) Change of colonic transit in vivo measured by bead expulsion time before and after TAM treatment ( n =10-11; * P <0.05; Students t -test). ( e ) Ex vivo muscle strip recordings showing spontaneous mechanical activity of ileal circular smooth musculature from TAM-treated control (upper panel) and c-Kit CreERT2/+ ; LSL-R26 DTA/+ animals (middle and lower panel, representative traces of two different animals). ( f ) Quantification of rhythmic contractions in e . The number of contractions with a regular distance between the peaks was counted (1 min of trace was analysed, n =11; *** P <0.001; Students t -test). Frequency ( g ) and calculated s.d. of amplitude ( h ) of contractions in ileum preparations (1 min trace of each animal was analysed, n =8-9; * P <0.05; Students t -test). ( i ) Intracellular microelectrode recordings display spontaneous electrical slow-wave activity in representative small intestinal circular smooth muscle cells from TAM-treated control animals (upper panel). Abolition of slow waves in TAM-treated c-Kit CreERT2/+ ; LSL-R26 DTA/+ mice (lower panel; n =3; recordings of 15 cells per animal). ( j ) Representative traces show contractile response of circular colonic muscle strips to EFS of TAM-treated control (upper left panel) and c-Kit CreERT2/+ ; LSL-R26 DTA/+ (lower left panel) mice. Right panel: graph showing EFS-induced contraction force relative to the baseline before EFS ( n =6-7; *** P <0.001; Students t -test). ( k ) Representative intracellular microelectrode recordings of colonic circular smooth muscle cells of the indicated genotypes in response to EFS ( n =3; recordings of 15 cells per animal). The EJP is lost in TAM-treated c-Kit CreERT2/+ ; LSL-R26 DTA/+ mice, whereas the fIJP and the sIJP remain unaffected by ICC depletion. All graphs show mean±s.e.m. Full size image ICC depletion blocks excitatory enteric neurotransmission There has been a long standing controversy whether ICC have a role in the regulation of excitatory and inhibitory neurotransmission, besides generating slow waves [8] , [9] , [10] , [11] , [12] , [13] , [14] , [15] , [16] , [26] . In small intestinal circular smooth muscle cells, ongoing slow waves with a frequency of ~30–35 cycles per min ( Fig. 3e ) typically mask neuronal-induced changes of electrical activity after electrical field stimulation (EFS; Supplementary Fig. S4b ). ICC-depleted animals lack slow-wave-type electrical activity in the small intestine; however, we did not observe EFS-induced changes of the membrane potential in circular smooth muscle cells ( Supplementary Fig. S4b ). Notably, we were not able to induce excitatory or inhibitory junction potentials (IJPs). ICC-depleted animals showed a marked and statistically significant depolarized resting membrane potential (RMP) in small intestinal circular smooth muscle cells (RMP c-Kit CreERT2/+ ; LSL-R26 DTA/+ +TAM: −52.9±3.7 mV versus RMP c-Kit CreERT2/+ +TAM (control): −62.4±3.0 mV; mean±s.e.m; n =6 animals per genotype; P <0.001, Students t -test; Figure 3i and Supplementary Fig. S4a,b ). This finding argues for a denervation of the smooth musculature from enteric neural input due to ICC depletion and is in accordance with previous reports showing a depolarized RMP in W/W v mice [7] . This depolarized RMP might be the electrical basis of the uncoordinated spontaneous contractions observed in the small intestine of ICC-depleted animals ( Fig. 3e ). In contrast to small intestine and in accordance with previous studies [27] , [28] , we did not observe slow-wave-type electrical activity and rhythmic contractions of colonic circular smooth muscle cells ( Fig. 3j–k and Supplementary Fig. S4c ). Therefore, intracellular recordings in the colon can be used to reliably study EFS-induced neurotransmission. To investigate excitatory intestinal neurotransmission in acute ICC-depleted adult animals, we measured neuronal-induced colonic contractions after EFS. Importantly, we observed a nearly complete blockade of excitatory neurotransmission as shown by strongly reduced contraction in response to EFS after ICC depletion ( Fig. 3j ). In line, ICC depletion completely abolished EFS-induced excitatory junction potentials (EJP) without affecting the IJP ( Fig. 3k ). In contrast to small intestine, the RMP was unaffected by ICC depletion in the colon (RMP c-Kit CreERT2/+ ; LSL-R26 DTA/+ +TAM: −57.3±4.2 mV versus RMP c-Kit CreERT2/+ +TAM (control): −60.6±2.7 mV; mean ±s.e.m; n =6 animals per genotype; not significant, Students t -test; Figure 3k ). These data provide the first genetic in vivo evidence for an essential role of ICC in excitatory neurotransmission to smooth muscle cells in acute ICC-depleted adult animals and support findings in W/W v germline mutant mice that display reduced excitatory neurotransmission and a hypotensive lower oesophageal and pyloric sphincter [12] , [13] , [16] , [29] , [30] . Deletion of Prkg1 blocks inhibitory neurotransmission To test whether ICC also modulate inhibitory neurotransmission to orchestrate GI motility, we deleted cGMP-dependent protein kinase I ( Prkg1 ) in ICC of adult animals by TAM administration using floxed Prkg1 mice ( Prkg1 f/f ). Prkg1 is a central mediator of the nonadrenergic, noncholinergic (NANC) neurotransmitters nitric oxide (NO) and carbon monoxide (CO), which are generated in enteric neurons by neuronal NO synthase (nNOS) and haem oxigenase, respectively [31] , [32] . Neuronal-derived NO and CO induces smooth muscle relaxation in the GI tract via activation of Prkg1 [32] , [33] , [34] . Accordingly, global Prkg1 -deficient mice (termed Prkg1 knock out (KO)) show a lack of NO-dependent smooth muscle relaxation associated with severe GI dysfunction [31] . Interestingly, inducible smooth muscle cell-specific deletion of Prkg1 in adult animals does not phenocopy global Prkg1 deficiency in the gut, indicating a possible role for an additional cell type in neuronal-induced smooth muscle relaxation. ICCs express the β-isoform of Prkg1 (termed PKG1β) in the small and large intestine ( Fig. 4a and Supplementary Fig. S5b ). TAM administration to c-Kit CreERT2/+ ; Prkg1 f/f animals resulted in recombination of the Prkg1 locus and loss of Prkg1 expression in only ~40% of all ICC ( Fig. 4c-e ). Nevertheless, we observed a profound GI motor dysfunction in mice with a partial deletion of Prkg1 in the ICC network, as evidenced by an increased GI transit time of ~2 h ( Fig. 4f ). It is well established that the network structure of ICC is essential for generation and propagation of slow waves as demonstrated in Fig. 3 (ref. 5 ). Here we show, in addition, that nitrergic neurotransmission via Prkg1 critically depends on the integrity of the ICC network. This might be also relevant for human GI motility disorders, where partial interruption of the ICC network has been described [35] . Importantly, slow-wave amplitude and rhythmicity was unaffected by Prkg1 deletion, as evidenced by normal ileal contractions ( Supplementary Fig. S5c-f ). However, we observed a moderate but significant change in the contraction frequency in TAM-treated c-Kit CreERT2/+ ; Prkg1 f/f animals ( Supplementary Fig. S5e ). This points to an additional, previously unrecognized role of Prkg1 in the modulation of slow-wave activity in vivo . 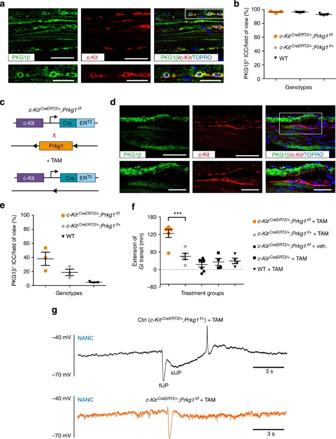Figure 4: ICC-specific deletion ofPrkg1blocks inhibitory neurotransmission. (a) Representative immunohistochemical analysis of c-Kit (red) and PKG1β (Prkg1β; green) expression in colon of WT animal. Nuclei are counterstained with TOPRO-3 (blue). Scale bars, 50 μm for micrographs, 25 μm for high-magnification panels. (b) Quantification of PKG1β (Prkg1β)-positive ICC in untreatedc-KitCreERT2/+;Prkg1flf,c-KitCreERT2/+;Prkg1f/+and WT animals (n=3 per group; 30 representative fields of view per mouse) shows similar numbers of double-positive ICC. (c) Genetic strategy used to deletePrkg1in ICC. (d) Representative confocal image of murine colon showing loss ofPrkg1(green) expression in c-Kit (red)-positive ICC after TAM treatment. Scale bars, 50 μm for micrographs, 25 μm for high-magnification panels. (e) Quantification of PKG1β (Prkg1β) expression in ICC of TAM-treated mice with the indicated genotypes. Deletion of PKG1β expression was observed in ~40% of all ICC inc-KitCreERT2/+;Prkg1f/fanimals after 3 days of TAM treatment (n=3 per group; 30 representative fields of view per animal). (f) Extension of whole GI transit time after 3 days of TAM or vehicle (veh.) treatment of the indicated genotypes (***P<0.001; Studentst-test). (g) Representative intracellular microelectrode recordings of colonic circular smooth muscle cells of the indicated genotypes in response to EFS under NANC conditions (n=3 per genotype; recordings of 15 cells per animal). sIJP is lost in TAM-treatedc-KitCreERT2/+;Prkg1f/fmice (lower panel) compared with TAM-treatedc-KitCreERT2/+;Prkg1f/+mice (upper panel). The fIJP remained unchanged. All graphs show mean ±s.e.m. Figure 4: ICC-specific deletion of Prkg1 blocks inhibitory neurotransmission. ( a ) Representative immunohistochemical analysis of c-Kit (red) and PKG1β (Prkg1β; green) expression in colon of WT animal. Nuclei are counterstained with TOPRO-3 (blue). Scale bars, 50 μm for micrographs, 25 μm for high-magnification panels. ( b ) Quantification of PKG1β (Prkg1β)-positive ICC in untreated c-Kit CreERT2/+ ; Prkg1 flf , c-Kit CreERT2/+ ; Prkg1 f/+ and WT animals ( n =3 per group; 30 representative fields of view per mouse) shows similar numbers of double-positive ICC. ( c ) Genetic strategy used to delete Prkg1 in ICC. ( d ) Representative confocal image of murine colon showing loss of Prkg1 (green) expression in c-Kit (red)-positive ICC after TAM treatment. Scale bars, 50 μm for micrographs, 25 μm for high-magnification panels. ( e ) Quantification of PKG1β (Prkg1β) expression in ICC of TAM-treated mice with the indicated genotypes. Deletion of PKG1β expression was observed in ~40% of all ICC in c-Kit CreERT2/+ ; Prkg1 f/f animals after 3 days of TAM treatment ( n =3 per group; 30 representative fields of view per animal). ( f ) Extension of whole GI transit time after 3 days of TAM or vehicle (veh.) treatment of the indicated genotypes (*** P <0.001; Students t -test). ( g ) Representative intracellular microelectrode recordings of colonic circular smooth muscle cells of the indicated genotypes in response to EFS under NANC conditions ( n =3 per genotype; recordings of 15 cells per animal). sIJP is lost in TAM-treated c-Kit CreERT2/+ ; Prkg1 f/f mice (lower panel) compared with TAM-treated c-Kit CreERT2/+ ; Prkg1 f/+ mice (upper panel). The fIJP remained unchanged. All graphs show mean ±s.e.m. Full size image Intracellular recordings in colonic circular smooth muscle cells showed that ICC-specific deletion of Prkg1 abolished specifically the NO-dependent nitrergic slow component of the IJP (sIJP) under NANC conditions ( Fig. 4g and Supplementary Fig. S5g ). This effect is again not mediated by mast cells as they lack expression of Prkg1 ( Supplementary Fig. S5a ). Addition of the NOS inhibitor L-N G -nitroarginine blocked specifically the sIJP in control animals ( c-Kit CreERT2/+ ; Prkg1 f/+ ), thus validating our results ( Supplementary Fig. S5g ). As expected, deletion of the NO-target Prkg1 in ICC showed no effect on ATP-dependent purinergic inhibitory neurotransmission, which is responsible for the fast and larger component of the IJP (fIJP; Fig. 4g and Supplementary Fig. S5g ). The mechanisms by which enteric neurons transmit their signals to regulate smooth muscle activity are of outstanding importance for basic and clinical science. The classical view of enteric neurotransmission to the smooth musculature is that enteric neurons release excitatory or inhibitory neurotransmitter that act directly on smooth muscle cells, thereby causing contraction or relaxation of the gut [9] . Functional analysis of ICC has provided crucial insights into the generation of pacemaking currents and slow-wave activity in the gut in health and disease [4] , [7] , [17] , [36] , [37] . However, because of the general lack of genetic studies targeting ICC or signalling pathways in ICC, it is still highly controversial whether ICC are involved in enteric neurotransmission [9] , [10] , [11] , [16] . These controversies are mainly because of the use of murine hypomorphic c-Kit germline mutants (like the W/W v model) in nearly all studies investigating ICC function [9] , [11] , [16] . The W/W v germline mutation severely impairs the c-Kit function, resulting in a reduced number or lack of specific ICC subpopulations, such as intramuscular ICC. However, this lack of ICC is region-specific and is already present during embryonic and postnatal development. Region and ICC subtype-specific effects, as well as developmental defects or compensatory mechanisms in these germline mutants, might affect smooth muscle function and neuromuscular transmission, resulting in contradictory findings [9] , [16] , [38] . In addition, currently used models do not allow inducible and selective genetic manipulation of a specific signalling pathway in ICC (target selectivity). As loss of ICC in W/W v mice may affect many different and opposing pathways, conclusions about the causative role of a specific pathway are therefore problematic. In this study, we developed a new mouse model to target ICC in vivo in adult animals at the genetic level by generation of a CreER T2 knock-in allele at the endogenous c-Kit locus. This model allows for the first time spatio-temporal genetic manipulation and lineage tracing of ICC in vivo . We found that acute TAM-induced depletion of ICC by conditional expression of DTA, or acute deletion of the NO/CO-cGMP target Prkg1 in ICC, impairs neurotransmission in the GI tract of adult animals. Depletion of ICC results in a specific loss of excitatory enteric neurotransmission as evidenced by the observed lack of EJPs and contractions in colonic smooth muscle cells. Unexpectedly, ICC depletion showed no effect on both components of the IJP, whereas disruption of NO/CO signalling in ICC by Prkg1 deletion blocks selectively the NO/CO-dependent sIJP. These findings are in line with data from mice lacking intramuscular ICC ( W/W v mice) or the gene encoding nNOS [29] , [30] . The lower oesophageal sphincter and the pyloric sphincter are hypotensive, with normal nitrergic relaxation in W/W v mice due to the selective lack of excitatory cholinergic input from enteric neurons (loss of EJP, unaffected IJP, for comparison see Fig. 3k ). In contrast, both sphincters are hypertensive in nNOS KO mice because of the selective lack of NO-dependent inhibitory innervation (loss of sIJP, for comparison see Fig. 4g ). These findings indicate that ICC, which express high amounts of Prkg1 (see Fig. 4a and ref. 39 ), are the primary target of NO released from enteric neurons. ICC are intercalated between enteric neurons and smooth muscle cells, and form close contacts with nitrergic nerve varicosities [13] , [26] . The release of neuronal-derived NO is spatially restricted, and NO targets only cells in close proximity to the releasing neuron. ICC, therefore, might act as scavengers to locally restrict NO signalling in the gut. Depletion of ICC could thus result in a spillover of NO to smooth muscle cells, thus inducing sIJP and smooth muscle relaxation in the absence of ICC. In contrast, deletion of Prkg1 in ICC does not affect this scavenger function, as the NO receptor soluble guanylyl cyclase is highly expressed in ICC [39] , [40] . Therefore, neuronally released NO can still bind and activate the NO receptor soluble guanylyl cyclase with a subsequent increase of cGMP levels in Prkg1 -deficient ICC; however, downstream NO–cGMP signalling is blocked by inactivation of the cGMP effector Prkg1 . Therefore, it is plausible that Prkg1 deletion in ICC, but not ICC depletion, inhibits sIJP and inhibitory neurotransmission from enteric neurons to smooth muscle cells. Whether the purinergic ATP-dependent fIJP is regulated via ICC remains an outstanding question, which has to be addressed by conditional loss-of-function experiments in the future. Data from W/W v mice indicate that the purinergic fIJP potential is not altered by the loss of ICC subpopulations [41] . Taken together, our results may explain and resolve the apparently contradictory findings in W/W v and nNOS KO models, which are the basis of the long-lasting controversy on how NO released from enteric neurons relaxes the smooth musculature [9] , [12] , [29] , [30] , [42] . The data presented in this manuscript demonstrate clearly that our novel Cre/loxP-based mouse model has several advantages compared with currently used animal models to study ICC in vivo . Time-specific acute interference with ICC function in adult animals in a cell-specific fashion, using the TAM-activatable Cre/loxP system, precludes adaptive and compensatory mechanisms or developmental defects of ICC and other cell types as the cause of the observed effects [9] , [11] . Importantly, by using adoptive bone marrow transfer experiments we can exclude a role of mast cells in our study, which have been suggested to have an important role in GI motility [43] . Therefore, the results of our study provide the first in vivo genetic evidence that acute impairment of ICC function results in a loss of excitatory and inhibitory neurotransmission in adult mice, and indicate that ICC link slow-wave activity with enteric neurotransmission in vivo . These findings support the concept that the core units that control GI motility are made up of nerves, ICC and smooth muscle cells [44] . In contrast to the central nervous system, enteric nerves utilize a second layer of regulation and integration to shape the functional output of nerve activity. This argues for a pivotal role of ICC in the organization and control of coordinated gut peristalsis beyond their role as GI pacemaker cells. Impairment of the ICC function causes severe GI motor disorders, which are believed to be due to the loss of slow-wave activity [4] , [7] , [17] . As ICC integrate slow-wave activity and enteric neurotransmission, the results of our study support the conclusion that these disorders are at least, in part, due to impaired neurotransmission. Materials All cell culture reagents were obtained from Invitrogen (Groningen, The Netherlands). Primers were made by MWG (Ebersberg, Germany) and restriction endonucleases were obtained from New England Biolabs (Mannheim, Germany). The E. coli strains TOP10 and Stbl3 (Invitrogen) were used for transformation and plasmid amplification. TAM-free base, Peanut oil, Atropine, Guanethidine, Nifedipine and L-N G -Nitroarginine were purchased from Sigma (Deisenhofen, Germany). Indocyanine green was purchased from Pulsion Medical Systems (Munich, Germany). Generation of the c-Kit CreERT2 mouse line Targeting the c-Kit locus by a knock-in strategy of CreER T2 into the ATG start codon of c-Kit was performed as previously described for the Rosa26 locus [45] . A targeting vector containing an frt-site-flanked neomycin resistance cassette 3′ of the CreER T2 (ref. 46 ) expression cassette was generated by standard cloning procedures ( Supplementary Fig. S1a ). The linearized targeting vector was electroporated into 129S6 embryonic stem (ES) cells. ES cells were selected with 200 μg ml −1 G418, and appropriately targeted clones were identified by PCR. Correct recombination and single-copy insertion was verified by Southern blot analysis with 32 P-labelled 5′- and 3′-external probe and internal probe, respectively, for the neomycin resistance cassette ( Supplementary Fig. S1b ). Twelve per cent of the analysed ES cell clones showed correct homologous recombination, and two clones (number 2 and number 5 in Supplementary Fig. S1b ) were injected into C57BL/6J blastocysts (Polygene, Rümlach, Switzerland). Germline transmission was achieved in two out of two clones, harbouring the targeted allele. A three-primer PCR strategy ( Supplementary Fig. S1c ) was used to genotype animals. Mouse strains R26 mT-mG/+ (ref. 19 ), LSL-R26 DTA/+ (ref. 20 ), conditional Prkg1 f/+ (ref. 47 ) and global Prkg1 KO (ref. 47 ) mice have been described previously. The strains were interbred with the c-Kit CreERT2/+ knock-in line to obtain compound mutant mice on a mixed C57Bl/6;129S6 background as previously described [48] . All animal studies were conducted in compliance with European guidelines for the care and use of laboratory animals, and were approved by the respective local authorities. Confocal laser-scanning microscopy Samples were examined by confocal laser-scanning microscopy (LSM) using a Zeiss LSM 510 Axiovert 100 microscope (Zeiss, Oberkochen, Germany) equipped with a × 20/0.5 air and a × 40/1.3 oil-immersion objective (optical section thickness 4.4 μm), or a Leica TCS SP5 DMI 6000 CS microscope equipped with a × 20/0.7 (optical section thickness 3 μm) and a × 40/1.25 (optical section thickness 1.5 μm) oil-immersion objective (Leica, Heidelberg, Germany). Images (single optical sections and z -stacks, z -step size 0.5 μm) with a frame size of 1,024 × 1,024 pixels and an image size of 225 × 225 μm (× 40/1.3 objective, Zeiss), 450 × 450 μm (× 20/0.5 air objective, Zeiss), 387.5 × 387.5 μm (× 40/1.25 objective, Leica) and 775 × 775 μm (× 20/0.7 objective, Leica) were collected. Images were merged and converted with Zeiss LSM 510 or Leica LAS AF software, respectively. Immunofluorescence staining Analysis of frozen sections was performed using murine tissue specimens fixed in 4% buffered formalin for 2 h, dehydrated in grade sucrose solutions at 4 °C (15% sucrose in PBS for 4 h followed by 30% sucrose overnight) and embedded in Miles Tissue-Tek (Sakura, Torrance, CA) before being rapidly frozen in liquid nitrogen. Frozen sections (20–30 μm thick) were obtained using a cryostat (Microm HM 560, Thermo Scientific, Schwerte, Germany). Briefly, slides were brought to room temperature (RT), fixed in 4% buffered formalin for 1 min, washed twice in PBS and incubated for 1 h in PBS containing 3% (w/v) bovine serum albumin (BSA), 1% (v/v) Triton-X 100 and 1% (w/v) saponin. Slides were incubated for at least 48 h at 4 °C with primary antibodies c-Kit (M14) (goat, 1:100; sc-1494, Santa Cruz Biotechnology, Santa Cruz, CA) and PKG1β (Prkg1β) (rabbit, 1:100) [49] . After rinsing, slides were incubated in the dark with secondary antibodies Alexa Fluor 594 donkey anti-goat or Alexa Fluor 488 chicken anti-rabbit (both 1:200; Invitrogen). The same protocol was used for double immunofluorescence staining. Nuclei were stained with TOPRO-3-iodide (1:1,000; Invitrogen) for 2 h in the dark at RT. After three rinses in PBS, slides were mounted with Vectashield Mounting Medium (Vector Laboratories, Burlingame, CA). For counting ICC, transversal sections of 3 animals of each genotype and 30 fields of view were analysed using the Zeiss LSM 510 microscope with the × 40/1.3 oil-immersion objective, and at least 2 different frozen sections (30 μm). For whole-mount preparations of colon and ileum, tissue specimens were flushed with PBS, opened along the mesenteric border, stretched out and mucosal side were pinned up flat on the surface of a Sylgard-coated petri dish. After removal of the mucosa using a Zeiss OPMI 1-FC stereomicroscope, tissues were fixed for 30 min in 4% buffered formalin and washed several times with PBS. For colonic tissue specimens, the submucosal plexus was dissected to ensure a better antibody penetration. The tissues were incubated in PBS containing 3% BSA for 1 h at RT, stained with primary antibodies as described above for at least 48 h at 4 °C with constant agitation, rinsed three times in PBS and then incubated for another 2 h in the dark at RT with secondary antibodies. Nuclear staining was achieved using TOPRO-3-iodide. For staining of skin mast cells, ears of the respective animals were separated into a ventral and dorsal half, and the half without cartilage was used. Tissues were fixed in 1% buffered formalin at 4 °C overnight. After incubation in 1% BSA in PBS for 1 h at RT, mast cells were stained with avidin–Texas Red (1:500; Invitrogen) as described previously [50] . Nuclei were counterstained with TOPRO-3-iodide. For mast cell counting, the ears of 3 mice per genotype and 15 fields of view of each animal were analysed using the Zeiss LSM 510 microscope with the × 20/0.5 air objective. Ex vivo GI motility studies The entire gut was removed and immediately placed in ice-cold Krebs solution (pH 7.4) containing (in mmol l −1 ): 117 NaCl, 4.7 KCl, 2.5 CaCl 2 (2H 2 O), 1.5 MgCl 2 (6H 2 O), 25 NaHCO 3 , 1.2 NaH 2 PO 4 and 11 glucose. The tissues were opened along the mesenteric border, thoroughly washed and mucosal side were pinned up in Sylgard-coated petri dishes, and full-thickness segments (1 cm) were cut along the circular muscle axis using an Olympus SZ30 stereomicroscope (Olympus, Hamburg, Germany). The segments of ileum and distal colon were mounted in individual 25-ml organ baths between two platinum electrodes and were maintained in oxygenated (95% O 2 , 5% CO 2 ) Krebs solution at 37 °C. Using a thread that was fixed at one end of each segment, the tissues were attached to an isometric tension transducer connected with a Quad Bridge and a MacLab/4S analogue/digital converter (MacLab, AD Instruments, Spechbach, Germany). Responses were recorded and analysed employing Chart 4.2 software (MacLab, AD Instruments). After mounting in the organ bath, tissues were equilibrated with a preload set at 15 mN for ~30 min. All tissues used in the experiments were vital and responded to EFS, which was performed at the beginning of each experiment using a Grass SD9 stimulator set at a constant supramaximal voltage of 100 V, 10 Hz with a pulse width of 0.6 ms for 10 s. The same conditions were used for following EFS. For investigating the rhythmicity of ileal muscle cell contractions, the trace of each animal was analysed by measuring the distance between single contraction peaks (3 × 1 min per animal, n =11). Furthermore, the frequency and s.d. of amplitude of ileal contractions was calculated (1 min per animal, n =8–9 animals of each genotype). Colon EFS-evoked responses were analysed by investigating the contraction force (6–7 animals of each genotype). Intracellular recordings Tissue preparation for electrophysiological experiments and intracellular recordings of smooth muscle cells of the circular muscle layer of mouse proximal colon and ileum were performed exactly as described previously [51] , [52] , [53] . Nifedipine (1 μM) was present throughout all experiments. Neurons were stimulated with single pulses (15 V, 0.3 ms duration) via a platinum electrode, arranged perpendicularly to the circular muscle layer, and connected to a Grass S11 stimulator via a stimulus isolation unit (Grass SIU59, Grass Instruments, Quincy, MA). EFS of the neurons caused changes in the RMP of the smooth muscle cells, and the responses were recorded against a ‘ground’ Ag-AgCl electrode placed in the bath medium. Evoked electrical events were amplified (DUO 733 microelectrode amplifier, World Precision Instruments, Sarasota, FL) and digitalized with an analogue-to-digital converter (SCB 68 interface, National Instruments, Austin, TX). Permanent recordings of membrane potentials were made using the LABVIEW 5.0 programme (National Instruments, Munich, Germany). For NANC measurements, 1 μM atropine and 1 μM guanethidine (both from Sigma) were used. The inhibitor of NOS L-N G -nitroarginine was added in a final concentration of 10 mM. Cells from three animals per genotype were analysed in all experiments. Statistical analyses Comparisons among data sets were made with analysis of variance, followed by Students t -test. A Bonferroni correction of the P -values was performed for multiple testing. Values of P <0.05 or less were considered to be statistically significant. How to cite this article: Klein, S. et al . Interstitial cells of Cajal integrate excitatory and inhibitory neurotransmission with intestinal slow-wave activity. Nat. Commun. 4:1630 doi: 10.1038/ncomms2626 (2013).